Selective inhibition of microRNA accessibility by RBM38 is required for p53 activity MicroRNAs (miRNAs) interact with 3′-untranslated regions of messenger RNAs to restrict expression of most protein-coding genes during normal development and cancer. RNA-binding proteins (RBPs) can control the biogenesis, stability and activity of miRNAs. Here we identify RBM38 in a genetic screen for RBPs whose expression controls miRNA access to target mRNAs. RBM38 is induced by p53 and its ability to modulate miRNA-mediated repression is required for proper p53 function. In contrast, RBM38 shows lower propensity to block the action of the p53-controlled miR-34a on SIRT1. Target selectivity is determined by the interaction of RBM38 with uridine-rich regions near miRNA target sequences. Furthermore, in large cohorts of human breast cancer, reduced RBM38 expression by promoter hypermethylation correlates with wild-type p53 status. Thus, our results indicate a novel layer of p53 gene regulation, which is required for its tumour suppressive function. Regulation of gene expression is a fundamental and multilayered process used by the cell to orchestrate or modulate organism development, homeostasis and environmental adaptation, among others. Each step involved in the pathway of gene expression, from RNA transcription to protein production, including pre-messenger RNA splicing and polyadenylation, as well as mRNA stability, transport and translation, is tightly controlled by a variety of protein and RNA effectors. MicroRNAs have recently gained attention owing to the magnitude of their influence on mRNA stability and protein translation. MicroRNAs are small non-coding RNAs able to direct translation repression, mRNA degradation, or a combination of the two [1] , [2] . Interestingly, bioinformatic predictions suggest that mammalian miRNAs could influence up to 60% of all protein-coding genes, supporting the importance of these non-coding RNA regulators [3] . Reflecting the broad impact of miRNAs on gene regulation, it is not surprising to find deregulation of miRNA expression in a variety of cancers as well as in some inflammatory, neurodegenerative and cardiovascular diseases [4] , [5] , [6] , [7] , [8] , [9] , [10] , [11] . Deregulation of miRNAs can occur through genetic alterations that can affect the production of the primary miRNA transcript, processing to mature miRNA, and influence miRNA–mRNA interaction [12] , [13] , [14] , [15] , [16] . Interestingly, an association has been established between colon cancer and two frameshift mutations in the TARBP2 gene, an RNA-binding protein regulating DICER stability and miRNA processing [17] . Both frameshifts introduce premature stop codons that produce a truncated dysfunctional TARBP2 that is unable to stabilize DICER, causing a lower miRNA production, and favouring tumorigenic growth. RNA-binding proteins (RBPs) have a fundamental role in posttranscriptional control of gene expression by regulating and coordinating the different processes of mRNA metabolism and translation [18] . One of the mechanisms used in this regulation is the modulation of miRNA production and activity. An example is the mechanism involving the RBP lin-28 and the miRNA let-7. By binding to the terminal loop of let-7 precursors, lin-28 interferes with the processing mediated by DGCR8 or Dicer, contributing to the maintenance of an undifferentiated state [19] , [20] , [21] , [22] . Additionally, miRNA activity can be enhanced or hindered by RBPs bound to target mRNA. For example, the RBP HuR binds to the 3′UTR of CAT-1 mRNA and relieves the miR-122 repression during different stress conditions [23] . Alternatively, the RBP pumilio binds to p27-3′UTR and induces a local change in RNA structure to favour the binding of miR-221 and miR-222 (ref. 24 ). Many stress conditions activate the tumour suppressor p53 to coordinate an adequate gene expression response. Interestingly, p53 function is partly mediated through the regulation of miRNAs and RBPs. During DNA damage, p53 interacts with both DGCR8 and DDX5 to enhance the processing of several miRNAs [25] . In addition, p53 directly activates the miR-34 family, which in turn interferes with the expression of several cell cycle and survival promoting genes [26] , [27] . The stress-activated p53 can also promote the induction of RBPs. For example, the double-stranded-RNA-binding zinc finger ZMAT3 is a direct target of p53 and is capable of binding p53-3′UTR, to increase its stability [28] . The RNA-binding protein RBM38 is also targeted by p53 and is required, by unknown mechanism, to efficiently induce p21 protein levels during stress conditions [29] . Here we report that RBM38 is required to decrease miRNA accessibility on a number of p53-induced transcripts, allowing an optimal target gene induction and cell cycle control. In contrast, RBM38 does not significantly affect the activity of miR-34a, a p53 target miRNA that is required for p53 function, on its target SIRT1. A combination of in vivo and in vitro binding assays, and mutational analysis, shows that binding of RBM38 to target 3′UTRs is essential to control the activity of specific miRNAs. Altogether, we propose that RBM38 supports p53 in initiating an efficient cellular stress response by selective blocking of miRNA action on different p53-induced mRNAs. A functional genetic screen to identify regulators of miRNAs To identify regulators of miRNA activity, we performed an RBP screen. We constructed an expression library of ∼ 100 RBPs ( Supplementary Table S1 ) and used as bait miR-150 and its target c-Myb-3′UTR cloned in the psiCHECK2 dual luciferase vector ( Fig. 1a ) [30] . We co-transfected c-Myb-3′UTR, the miR-150 or the control miR-206 with the RBP library into U2OS cells and calculated the impact of miR-150 on Renilla /Firefly luciferase ratios ( Fig. 1b ). Control transfections (red) showed the expected 2–2.5-fold reduction in gene expression by miR-150, and ectopic expression of Dnd1 (green) blocked miRNA effect, as reported previously [31] . For validation, we selected 8 RBPs that presented the most significant inhibitory effect on miR-150 function, but could confirm only RBM38 ( Fig. 1c ). 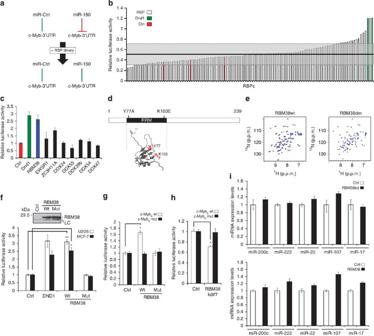Figure 1: RBM38 counteracts miR-150-mediated repression of c-Myb-3′UTR. (a) Screen illustration. U2OS cells were transfected with psiCHECK2-c-Myb-3′UTR, the control miR-206 or miR-150 construct. The RBP library was then transfected and relativerenilla/firefly levels were assessed 48 h later. (b) RBPs were plotted according to their miR-150/miR-206 ratios. Positive (green) and negative (red) controls as well as the mean (black line) ±s.d. (shaded area) are displayed. (c) Screen validation using same settings as in (a). The relative luciferase signals derived from the miR-150/miR-206 ratios were normalized to the control reaction and the latter was arbitrarily set to 1. RBM38 is shown in blue. Error bars represent standard deviation of technical replicates,n=3. (d) Secondary structure of the human RBM38 RRM domain. The residues Y77 and K103, which are mutated in RBM38mut, are displayed in red. (e) Overlay of15N1H correlation spectra recorded during the titration of wild-type (left panel) and mutant (right panel) RBM38 with an 5′-UUUUUU-3′ (U6) RNA oligo at 27 °C. Spectra are recorded at protein:RNA ratio of 1:0 (red), 1:1 (purple) and 1:3 (blue). (f) U2OS and MCF-7 cells were co-transfected with the indicated plasmids as in (a) and the luciferase signals were processed as in (c). Protein levels of RBM38 wild type and mutant are also shown. (g) U2OS cells were transfected with either the wild-type or the mutant c-Myb-short-3′UTR (c-Mybs-wt or c-Mybs-mut) and the indicated plasmids. The luciferase signals were processed as in (c). (h) U2OS cells were transfected with the reporters mentioned in (g) together with a control or a knockdown against RBM38. The luciferase signals were processed as in (c). (i) The level of various mature miRNAs was measured in U2OS cells transfected with scrambled siRNA (Ctrl) or siRNA against RBM38 (upper panel) and with an empty vector (Ctrl) or RBM38 expression vector (lower panel). GAPDH levels were used as an internal control for normalization. Error bars represent standard deviation of technical replicates,n=3. Data in (f,g,h) are representative of three independent experiments (mean±s.d., *P<0.05; **P<0.005, two-tailed student'st-test). Figure 1: RBM38 counteracts miR-150-mediated repression of c-Myb-3′UTR. ( a ) Screen illustration. U2OS cells were transfected with psiCHECK2-c-Myb-3′UTR, the control miR-206 or miR-150 construct. The RBP library was then transfected and relative renilla /firefly levels were assessed 48 h later. ( b ) RBPs were plotted according to their miR-150/miR-206 ratios. Positive (green) and negative (red) controls as well as the mean (black line) ±s.d. (shaded area) are displayed. ( c ) Screen validation using same settings as in ( a ). The relative luciferase signals derived from the miR-150/miR-206 ratios were normalized to the control reaction and the latter was arbitrarily set to 1. RBM38 is shown in blue. Error bars represent standard deviation of technical replicates, n =3. ( d ) Secondary structure of the human RBM38 RRM domain. The residues Y77 and K103, which are mutated in RBM38mut, are displayed in red. ( e ) Overlay of 15 N 1 H correlation spectra recorded during the titration of wild-type (left panel) and mutant (right panel) RBM38 with an 5′-UUUUUU-3′ (U6) RNA oligo at 27 °C. Spectra are recorded at protein:RNA ratio of 1:0 (red), 1:1 (purple) and 1:3 (blue). ( f ) U2OS and MCF-7 cells were co-transfected with the indicated plasmids as in ( a ) and the luciferase signals were processed as in ( c ). Protein levels of RBM38 wild type and mutant are also shown. ( g ) U2OS cells were transfected with either the wild-type or the mutant c-Myb-short-3′UTR (c-Myb s -wt or c-Myb s -mut) and the indicated plasmids. The luciferase signals were processed as in ( c ). ( h ) U2OS cells were transfected with the reporters mentioned in ( g ) together with a control or a knockdown against RBM38. The luciferase signals were processed as in ( c ). ( i ) The level of various mature miRNAs was measured in U2OS cells transfected with scrambled siRNA (Ctrl) or siRNA against RBM38 (upper panel) and with an empty vector (Ctrl) or RBM38 expression vector (lower panel). GAPDH levels were used as an internal control for normalization. Error bars represent standard deviation of technical replicates, n =3. Data in ( f , g , h ) are representative of three independent experiments (mean±s.d., * P <0.05; ** P <0.005, two-tailed student's t -test). Full size image Interplay between RBM38 and miRNAs RBM38 contains one RNA recognition motif (RRM) domain. We, therefore, examined whether the miRNA-related function of RBM38 is dependent on the RNA-binding activity of its RRM domain by mutating two evolutionary conserved residues, Y77 and K103 ( Fig. 1d ) that are involved in canonical RRM–RNA binding [32] . In vitro NMR assays show that the Y77A/K103E mutant is folded and non-aggregated and that, in contrast to RBM38wt, does not bind to RNA ( Fig. 1e ; Supplementary Fig. S1 ). Overexpression of RBM38mut in both U2OS and MCF-7 cells did not affect miR-150 activity, whereas RBM38wt diminished miR-150 function ( Fig. 1f ). Thus, binding to RNA is required by RBM38 to inhibit miR-150 activity. Interestingly, like Dnd1 (ref. 31 ), RBM38 function was connected to miRNAs. When we mutated c-Myb-3′UTR in the miR-150 target sequences (c-Myb-short-mut-3′UTR or c-Myb s -mut-3′UTR), no regulation by RBM38 was observed ( Fig. 1g ; Supplementary Fig. S2 ). Moreover, transfection of an efficient short hairpin RNA (shRNA) against RBM38 ( Fig. 1h ; Supplementary Fig. S3 ) enhanced the inhibition mediated by miR-150 on c-Myb s -wt-3′UTR. This effect was specific and miRNA-related, as no significant effect was seen on c-Myb s -mut reporter ( Fig. 1h ). Of note, both the overexpression and knockdown of endogenous RBM38 were not associated with significant changes in mature miRNA expression and localization ( Fig. 1i ; Supplementary Figs S4 and S5 ). However, the effect of RBM38 was not restricted to miR-150/c-Myb-3′UTR, as the miR-206-mediated repression of Cx43-3′UTR was equally responsive to RBM38 ( Supplementary Fig. S6 ). Altogether, our results are consistent with a model whereby binding of RBM38 to target mRNAs restricts miRNA accessibility. RBM38, cellular stress and cell cycle RBM38 levels were shown to increase following DNA damage through p53, an effect that is required for p21 stimulation and cell cycle arrest [29] . Indeed, in MCF-7, U2OS and ZR-75.1 cells, RBM38 mRNA levels increased 2–3-fold in 24 h following doxorubicin treatment ( Fig. 2a ). This effect was diminished in cells transfected with a p53kd vector ( Fig. 2b ). Moreover, the expression of endogenous RBM38 was required to maintain normal levels of p21 in cycling cells, and induced high levels of p21 in DNA-damaged cells. 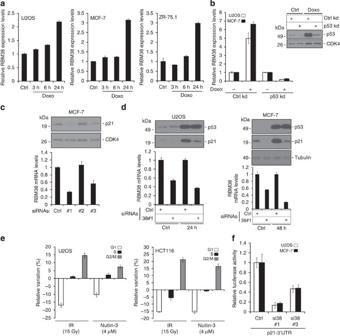Figure 2: RBM38 is induced by p53 and is required to sustain p21 levels. (a) Three different p53wt cell lines (U2OS, MCF-7 and ZR-75.1) were treated with 0.4 μg ml−1of doxorubicin (3, 6 and 24 h) and RBM38 mRNA levels were measured using RT–qPCR analysis. (b) RBM38 mRNA levels in stable cell lines transduced with control vector (Ctrl kd) or an shRNA-expressing vector against p53 (p53kd) were measured by RT–qPCR. An immunoblot assessing p53kd efficiency in U2OS under normal and stress (0.4 μg ml−1doxorubicin for 24 h) conditions is shown. (c) MCF-7 cells were transfected with a scramble (Ctrl) or 3 different siRNAs against RBM38. p21 and RBM38 levels were, respectively, measured using immunobloting, and RT–qPCR. CDK4 protein levels were used as a loading control. (d) MCF-7 and U2OS cells were transfected with scrambled siRNA (Ctrl) or siRNA against RBM38. p53, p21 and tubulin protein levels were visualized by immunoblot wheras RBM38 levels were quantified by RT–qPCR. (e) Cell-cycle-distribution change of U2OS and HCT116 cells transfected with scrambled siRNA or siRNA against RBM38 and treated with either ionizing radiation (15 Gy) or Nutlin-3 for 24 h. To capture cycling cells in G2/M, cells were incubated 12 h with nocodazol before flow cytometric analysis. (f) The p21-3′UTR reporter was co-transfected with scrambled siRNA (Ctrl) or 2 effective siRNAs against RBM38. The relative luciferase activity is presented as therenilla/firefly ratio normalized to the scramble reaction. Error bars in (a–f) represent standard deviation of technical replicates,n=3. First, Figure 2c shows that inhibition of RBM38 expression by two effective small interfering RNAs (siRNAs) reduced p21 protein levels. Second, loss-of RBM38 expression hampered the accumulation of p21 following DNA damage inflicted by doxorubicin in MCF-7 and U2OS cells ( Fig. 2d ). This, importantly, was despite normal induction of p53. Figure 2: RBM38 is induced by p53 and is required to sustain p21 levels. ( a ) Three different p53wt cell lines (U2OS, MCF-7 and ZR-75.1) were treated with 0.4 μg ml −1 of doxorubicin (3, 6 and 24 h) and RBM38 mRNA levels were measured using RT–qPCR analysis. ( b ) RBM38 mRNA levels in stable cell lines transduced with control vector (Ctrl kd) or an shRNA-expressing vector against p53 (p53kd) were measured by RT–qPCR. An immunoblot assessing p53kd efficiency in U2OS under normal and stress (0.4 μg ml −1 doxorubicin for 24 h) conditions is shown. ( c ) MCF-7 cells were transfected with a scramble (Ctrl) or 3 different siRNAs against RBM38. p21 and RBM38 levels were, respectively, measured using immunobloting, and RT–qPCR. CDK4 protein levels were used as a loading control. ( d ) MCF-7 and U2OS cells were transfected with scrambled siRNA (Ctrl) or siRNA against RBM38. p53, p21 and tubulin protein levels were visualized by immunoblot wheras RBM38 levels were quantified by RT–qPCR. ( e ) Cell-cycle-distribution change of U2OS and HCT116 cells transfected with scrambled siRNA or siRNA against RBM38 and treated with either ionizing radiation (15 Gy) or Nutlin-3 for 24 h. To capture cycling cells in G2/M, cells were incubated 12 h with nocodazol before flow cytometric analysis. ( f ) The p21-3′UTR reporter was co-transfected with scrambled siRNA (Ctrl) or 2 effective siRNAs against RBM38. The relative luciferase activity is presented as the renilla /firefly ratio normalized to the scramble reaction. Error bars in ( a – f ) represent standard deviation of technical replicates, n =3. Full size image Next, we examined the role of RBM38 in enforcing proper cell cycle checkpoints in response to DNA damage. We analysed expression profiles in control and RBM38kd MCF-7 cells that were incubated with and without doxorubicin for 24 h. Although a large portion of the transcriptional response to doxorubicin was not affected by knocking down RBM38, a major cluster of more than 100 genes was downregulated in response to doxorubicin in control, but not in RBM38kd cells ( Supplementary Fig. S7 ). Importantly, this cluster was significantly enriched for cell-cycle-related genes ( Supplementary Table S2 ). The downregulation of these genes reflects the strong activation of cell cycle arrest in response to the DNA damage-associated stress in the control cells, as well as the defect in this response when RBM38 expression is suppressed. We also observed that knocking down RBM38 undermines the activation of cell cycle arrest in response to genotoxic stresses. As shown in Figure 2e and Supplementary Figure S8a , inhibition of RBM38 expression in U2OS and HCT116 cells treated with ionizing radiation or Nutlin-3, resulted in a reduction of ∼ 10–15% of the G1-arrested cells. Similar results were also achieved with 3 different siRNAs against RBM38 ( Supplementary Fig. S8b,c ). Last, to examine whether the effect of RBM38 on p21 expression was mediated through p21-3′UTR, we cloned the p21-3′UTR downstream of Renilla luciferase in the psiCHECK2 vector. Co-transfection experiments with two effective RBM38 siRNAs showed that most, if not all, of RBM38 effect on p21 was mediated through the p21-3′UTR ( Fig. 2f ). Thus, our results confirm that RBM38 is a downstream target of p53 required for maintaining p21 protein levels during normal proliferation and following genotoxic stress through the p21-3′UTR. RBM38 blocks miRNA-mediated repression of p53 target genes Our results, thus far, suggest that RBM38 induces gene expression by inhibiting miRNA activity on target 3′UTRs. Particularly, p53-dependent maintenance of high-p21-protein level following DNA damage requires RBM38. These observations raised two issues: does RBM38 counteract the miRNA-mediated repression of diverse p53 target genes? ; how specific is the function of RBM38? To address the first question, we examined the effect of RBM38 overexpression and knockdown on the 3′UTR of several known direct transcriptional targets of p53 ( Fig. 3a ). Similar to the p21-3′UTR, RBM38wt induced the expression of Renilla luciferase when conjugated with the 3′UTRs of RBM38 itself, PCNA, DDIT4, TNFRSF10B, LATS2 and IER5 ( Fig. 3b ). Similarly, knocking down RBM38 affected the vast majority of these 3′UTRs ( Fig. 3c ). This indicates that RBM38 broadly functions to assist p53 in inducing its target genes. However, we also noticed that RBM38 function is not limited to p53-target genes ( Supplementary Fig. S9 ). To examine if this function is miRNA-dependent ( Fig. 3d ), we identified a few miRNAs that are able to repress RBM38, p21, DDIT4 and LATS2 ( Supplementary Fig. S10 ). In all cases, miRNA-mediated repression was largely counteracted by RBM38 overexpression ( Fig. 3e ). These results suggest that RBM38 helps to maintain the expression of p53 target genes, at least in part, by inhibiting targeting miRNAs. 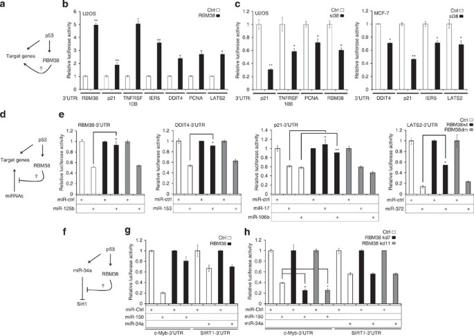Figure 3: Selective inhibition of miRNA activity by RBM38. (a) A scheme showing a hypothetical influence of RBM38 on p53 target genes. (b) Cells were co-transfected with various 3′UTR reporters of known direct transcriptional targets of p53 and RBM38wt (RBM38) or RBM38mut (Ctrl) expression vectors. The relative luciferase activities (renilla/firefly ratios) were normalized to RBM38mut reaction and the latter was arbitrarily set to 1. *P<0.05 and **P<0.005 (two-tailed student'st-test,n=3). (c) Cells were co-transfected with the 3′UTR reporters used in (b), together with either a scrambled (Ctrl) or RBM38 siRNA (si38). The relative luciferase activities (renilla/firefly ratios) were normalized to the control reaction. *P<0.05 and **P<0.005 (two-tailed student'st-test,n=3). (d) A model linking RBM38 function to miRNA blocking. (e) Cells were co-transfected with RBM38wt, RBM38mut expression vectors or an empty vector (Ctrl) and the indicated reporter/miRNAs. For each set, the relative luciferase activities (renilla/firefly ratios) were normalized to the miR-Ctrl reactions, and the latter were arbitrarily set to 1. *P<0.05 and **P<0.005 (two-tailed student'st-test,n=3). (f) Model addressing RBM38 specificity. (g) Cells were co-transfected with the indicated constructs together with RBM38 expression vector. An empty vector was used as control (Ctrl). All reactions were normalized as in (e). (h) Cells were co-transfected with the indicated constructs together with RBM38 knockdown vectors or a non-targeting shRNA (Ctrl). *P<0.05 (two-tailed student'st-test,n=3). Error bars in (b,c,e,g,h) represent standard deviation of technical replicates,n=3. Figure 3: Selective inhibition of miRNA activity by RBM38. ( a ) A scheme showing a hypothetical influence of RBM38 on p53 target genes. ( b ) Cells were co-transfected with various 3′UTR reporters of known direct transcriptional targets of p53 and RBM38wt (RBM38) or RBM38mut (Ctrl) expression vectors. The relative luciferase activities ( renilla /firefly ratios) were normalized to RBM38mut reaction and the latter was arbitrarily set to 1. * P <0.05 and ** P <0.005 (two-tailed student's t -test, n =3). ( c ) Cells were co-transfected with the 3′UTR reporters used in ( b ), together with either a scrambled (Ctrl) or RBM38 siRNA (si38). The relative luciferase activities ( renilla /firefly ratios) were normalized to the control reaction. * P <0.05 and ** P <0.005 (two-tailed student's t -test, n =3). ( d ) A model linking RBM38 function to miRNA blocking. ( e ) Cells were co-transfected with RBM38wt, RBM38mut expression vectors or an empty vector (Ctrl) and the indicated reporter/miRNAs. For each set, the relative luciferase activities ( renilla /firefly ratios) were normalized to the miR-Ctrl reactions, and the latter were arbitrarily set to 1. * P <0.05 and ** P <0.005 (two-tailed student's t -test, n =3). ( f ) Model addressing RBM38 specificity. ( g ) Cells were co-transfected with the indicated constructs together with RBM38 expression vector. An empty vector was used as control (Ctrl). All reactions were normalized as in ( e ). ( h ) Cells were co-transfected with the indicated constructs together with RBM38 knockdown vectors or a non-targeting shRNA (Ctrl). * P <0.05 (two-tailed student's t -test, n =3). Error bars in ( b , c , e , g , h ) represent standard deviation of technical replicates, n =3. Full size image Specificity of RBM38 function Beyond activating protein-coding genes, p53 also enhances miRNA processing in general [25] and activates miR-34a in particular [26] . This raises the question of specificity, as the induction of RBM38 may block p53-mediated miR-34a function. To address this issue, we examined SIRT1, a prominent and biologically relevant miR-34a target ( Fig. 3f ). Indeed, transfection of miR-34a inhibited SIRT1-3′UTR expression, but not c-Myb-3′UTR ( Supplementary Fig. S11 ). However, in contrast to the direct p53-target genes examined above, RBM38 overexpression had no significant effect on the repression of SIRT1-3′UTR by miR-34a ( Fig. 3g ). Moreover, RBM38 did not influence the levels of miR-34a ( Supplementary Fig. S12 ). Similar results were also obtained with FOXP1-3′UTR, another target of the miR-34a ( Supplementary Fig. S13 ). Conversely, loss-of RBM38 induces miR-150-mediated inhibition of c-Myb-3′UTR, while no effects were observed on miR-34a-mediated inhibition of SIRT1-3′UTR ( Fig. 3h ). These experiments show that RBM38 exhibits, to some extent, target specificity. To uncover the molecular mechanism underlying RBM38-selective inhibition of miRNA activity, we mapped RBM38-binding sites in HeLa cells by iCLIP [33] . Statistical analysis revealed that RBM38 binds preferentially to 3′UTRs ( Supplementary Fig. S14a ). The distribution of target sites along the 3′UTR was not even, as a greater occupancy was observed at the beginning and at the end of the 3′UTRs ( Supplementary Fig. S14b ). This pattern is similar to the miRNA binding profile and therefore suggested a relation between miRNA and RBM38 binding to the mRNA [34] . Intersection with the expression dataset detected a mild but statistically significant repression of the targets bound by RBM38 in the knocked-down samples ( Supplementary Fig. S14c ). De-novo motif discovery analysis revealed that, RBM38 is most often found bound to uridine-rich RNA regions (URRs) ( Supplementary Fig. S14d ). Supporting this observation, in vitro binding assays also demonstrated that RBM38 RRM binds with high affinity to polyU RNA oligos ( Fig. 1e ). Interestingly, although the two miR-150-binding sites in the c-Myb-3′UTR contained URRs, the equivalent region on SIRT1-3′UTR (miR-34a-binding sites), did not. This suggests that the presence of URRs in the vicinity of miRNA target sites determines target selectivity of RBM38 in our functional assays. To study in more detail the RBM38 interaction region on the 3′UTRs, we replaced the two miR-150-binding sites in c-Myb-3′UTR with the miR-34a sites of SIRT1-3′UTR ( Fig. 4a ; Supplementary Fig. S2 ). As expected, overexpression of miR-34a repressed c-Myb s -34a-3′UTR reporter, while overexpression of miR-150 inhibited c-Myb s -wt-3′UTR. Consistently, ectopic expression of RBM38wt completely diminished miR-150 function on the c-Myb s wt-3′UTR, but had only a slight effect on the miR-34a-mediated repression of the c-Myb s 34a-3′UTR ( Fig. 4b ). Inversely, replacing the two miR-34a-binding sites in the SIRT1 s -3′UTR ( Fig. 4a ; Supplementary Fig. S2 ) with the miR-150 sites of the c-Myb-3′UTR, increased the SIRT1 s -3′UTR sensitivity to RBM38 function ( Fig. 4c ). To directly link functional specificity to RRM–RNA binding, we measured the affinity of the RBM38 RRM domain for the miR-150 and miR-34a sites on the c-Myb-3′UTR and SIRT1-3′UTR, respectively. In vitro NMR assays showed that the in vivo target RNAs bind with substantially higher affinity than the non-target ones ( Supplementary Fig. S15 and Supplementary Table S3 ). One important question is, if recognition of p21, which is targeted by RBM38, but only has a short U stretch sequence compared with c-Myb (albeit it does contain U/G-rich stretches, like c-Myb), is mediated by the RRM domain. To answer this, we tested RBM38 RRM affinity for the miRNA seed site on the p21-3′UTR and compared this affinity with the one obtained for the SIRT1 and c-Myb RNAs. RBM38 binds to p21 with an affinity similar to the binding to c-Myb, which is substantially stronger than SIRT1, confirming a direct link between RRM–RNA binding and target specificity ( Fig. 4d and Supplementary Fig. S15 ) and showing that the iCLIP data, although consistent with our affinity measurements and, in general, with the observed in vivo targeting, are not strictly predictive. 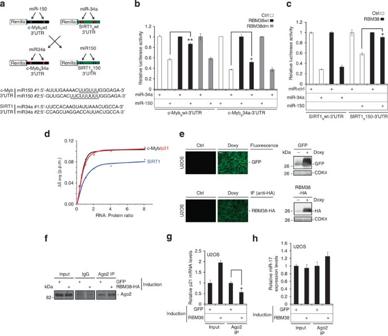Figure 4: RBM38 binds to u-rich regions and protects UTRs from Ago2-mediated repression. (a) Cartoon illustrating the luciferase reporter of c-Mybswt, SIRT1swt, c-Mybs34a and SIRT1s150-3′UTRs. Also shown are the miR-150-binding sites in c-Myb-3′UTR (blue boxes) and miR-34a-binding sites in SIRT1-3′UTR (red boxes). Putative RBM38-binding sites (u-rich stretches) are underlined in both miR-150-binding sites. (b) MCF-7 cells were co-transfected with c-Mybswt- or c-Mybs34a-3′UTR reporter and the indicated miRNAs. For each condition, the relative luciferase activities were normalized to the non-targeting miRNA reactions (*P<0.05 and **P<0.005, two-tailed student'st-test,n=3). (c) U2OS cells were co-transfected with SIRT1swt- or SIRT1s150-3′UTR reporter and the indicated miRNAs. For each condition, the relative luciferase activities were normalized to the non-targeting miRNA reactions (*P<0.05, two-tailed student'st-test,n=3). (d) Binding of RBM38wt to c-Myb, p21 and SIRT1 RNA oligos. The averaged chemical shift changes (Δδ of the V80 amide NH resonance on addition of the three RNAs are plotted against the RNA:protein ratio and the calculated binding curves are displayed in black (c-Myb), red (p21) and blue (SIRT1). (e) Tet-On system driving the GFP or RBM38-HA expression with doxycycline (1 μg ml−1for 24 h) treatment. Protein levels of both GFP and RBM38-HA were monitored by fluorescence/immunofluorescence (anti-HA) and immunoblotting (anti-GFP and anti-HA). CDK4 was used as a loading control. Scale bar 200 μM. (f) Immunoprecipitation of Ago2 in GFP- and RBM38-HA-induced (Doxy 1 μg ml−1for 24 h) U2OS cells. Cells were treated 12 h with Nutlin-3 (8 μM) before collecting. Protein levels of Ago2 in the input, control IP (IgG) and specific IP (Ago2 IP) were visualized by immunoblotting. (g) Measurement of p21 mRNA levels recovered from the Ago2 IP performed in (f). *P<0.05 (two-tailed student'st-test,n=3). (h) Measurement of miR-17 levels recovered from the Ago2 IP performed in (f). Error bars in (b,c,g,h) represent standard deviation of technical replicates,n=3. Figure 4: RBM38 binds to u-rich regions and protects UTRs from Ago2-mediated repression. ( a ) Cartoon illustrating the luciferase reporter of c-Myb s wt, SIRT1 s wt, c-Myb s 34a and SIRT1 s 150-3′UTRs. Also shown are the miR-150-binding sites in c-Myb-3′UTR (blue boxes) and miR-34a-binding sites in SIRT1-3′UTR (red boxes). Putative RBM38-binding sites (u-rich stretches) are underlined in both miR-150-binding sites. ( b ) MCF-7 cells were co-transfected with c-Myb s wt- or c-Myb s 34a-3′UTR reporter and the indicated miRNAs. For each condition, the relative luciferase activities were normalized to the non-targeting miRNA reactions (* P <0.05 and ** P <0.005, two-tailed student's t -test, n =3). ( c ) U2OS cells were co-transfected with SIRT1 s wt- or SIRT1 s 150-3′UTR reporter and the indicated miRNAs. For each condition, the relative luciferase activities were normalized to the non-targeting miRNA reactions (* P <0.05, two-tailed student's t -test, n =3). ( d ) Binding of RBM38wt to c-Myb, p21 and SIRT1 RNA oligos. The averaged chemical shift changes (Δδ of the V80 amide NH resonance on addition of the three RNAs are plotted against the RNA:protein ratio and the calculated binding curves are displayed in black (c-Myb), red (p21) and blue (SIRT1). ( e ) Tet-On system driving the GFP or RBM38-HA expression with doxycycline (1 μg ml −1 for 24 h) treatment. Protein levels of both GFP and RBM38-HA were monitored by fluorescence/immunofluorescence (anti-HA) and immunoblotting (anti-GFP and anti-HA). CDK4 was used as a loading control. Scale bar 200 μM. ( f ) Immunoprecipitation of Ago2 in GFP- and RBM38-HA-induced (Doxy 1 μg ml −1 for 24 h) U2OS cells. Cells were treated 12 h with Nutlin-3 (8 μM) before collecting. Protein levels of Ago2 in the input, control IP (IgG) and specific IP (Ago2 IP) were visualized by immunoblotting. ( g ) Measurement of p21 mRNA levels recovered from the Ago2 IP performed in ( f ). * P <0.05 (two-tailed student's t -test, n =3). ( h ) Measurement of miR-17 levels recovered from the Ago2 IP performed in ( f ). Error bars in ( b , c , g , h ) represent standard deviation of technical replicates, n =3. Full size image RBM38 restricts Ago2 accessibility to p21 mRNA Mechanistically, we hypothesized that RBM38 could interfere with miRNA function by binding to target mRNAs and preventing miRNA accessibility. To test this, we generated a Tet-On inducible system for RBM38-HA in U2OS cells. Figure 4e shows the induction of GFP and RBM38-HA in this system. We subsequently treated both induced cell lines with Nutlin-3, IPed Ago2 ( Fig. 4f ) and RBM38-HA, and examined their interaction with p21 mRNA. As expected, we found p21 mRNA bound to RBM38-HA ( Supplementary Fig. S16 ). In contrast, lower p21 mRNA levels were detected in Ago2 IPs from RBM38-induced cells ( Fig. 4g ). Moreover, as shown in Figure 4h , Ago2-bound miRNA-17 levels remain stable with RBM38 induction. Altogether, these results strongly support RBM38's function in binding to mRNAs and restricting miRNA accessibility. RBM38 function is linked to miRNA To further assess the connection between RBM38 and miRNAs, we overexpressed RBM38 in HCT116 wild type and in HCT116 dicer exon 5 knockout (ex5−/−) cells. 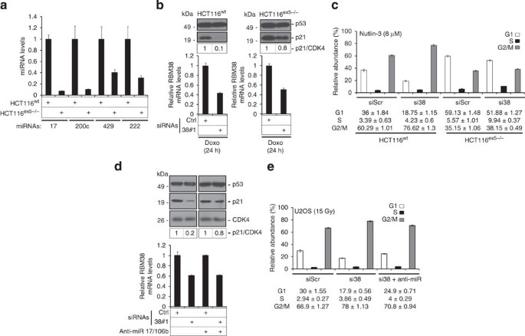Figure 5: miRNAs are required for efficient RBM38 effect on p21 and cell cycle. (a) Differential expression levels of miRNAs in HCT116wtand HCT116ex5−/−cell lines. The abundance of each indicated miRNA was measured by real-time qPCR using specific Taqman probes. miRNA levels in HCT116wtwere arbitrarily set to 1. (b) HCT116wtand HCT116ex5−/−cells were transfected with scrambled siRNA (Ctrl) or siRNA against RBM38 (38#1), treated with doxorubicin, and immunoblotted with anti-p21 and anti-p53 antibodies. Relative p21 protein levels were measured using the ImageJ software and RBM38 RNA levels were assessed by RT–qPCR. (c) Cell cycle analysis of HCT116wtand HCT116ex5−/−cells transfected with scrambled siRNA (siScr) or siRNA against RBM38 (si38), and treated with Nutlin-3. For the last 12 h, cells were incubated with nocodazol to capture cycling cells in G2/M. For each condition, the percentage of cells in each phase (G1-S-G2/M) is indicated. (d) U2OS cells were co-transfected with the indicated siRNAs, either with a control anti-miRNA or a specific anti-miR-17/106b pool and analysed as in panel (b). (e) Cell cycle analysis of U2OS cells transfected as in (d) and treated with ionizing radiation. Flow cytometry analysis was performed as in (c). All error bars in (a–e) represent standard deviation of technical replicates,n=3. As shown in Figure 5a , the levels of mature miRNAs are substantially lower in the HCT116 ex5−/− cells compared with HCT116 wt . We then postulated that knocking down RBM38 should preferentially reduce p21 protein levels in HCT116 wt , where the ratio miRNAs/RBM38 is high. Indeed, knocking down RBM38 in HCT116 wt cells resulted in a marked reduction in p21 activation following DNA damage treatment, while p21 was still accumulating in HCT116 ex5−/− ( Fig. 5b ). Remarkably, the induction of p21 in RBM38-knocked down HCT116 ex5−/− cells was prevented by the addition of the miR-17 duplex ( Supplementary Fig. S17 ). This suggests that a substantial part of the regulation of p21 by RBM38 is carried out through derepression of targeting miRNA activity. Figure 5: miRNAs are required for efficient RBM38 effect on p21 and cell cycle. ( a ) Differential expression levels of miRNAs in HCT116 wt and HCT116 ex5−/− cell lines. The abundance of each indicated miRNA was measured by real-time qPCR using specific Taqman probes. miRNA levels in HCT116 wt were arbitrarily set to 1. ( b ) HCT116 wt and HCT116 ex5−/− cells were transfected with scrambled siRNA (Ctrl) or siRNA against RBM38 (38#1), treated with doxorubicin, and immunoblotted with anti-p21 and anti-p53 antibodies. Relative p21 protein levels were measured using the ImageJ software and RBM38 RNA levels were assessed by RT–qPCR. ( c ) Cell cycle analysis of HCT116 wt and HCT116 ex5−/− cells transfected with scrambled siRNA (siScr) or siRNA against RBM38 (si38), and treated with Nutlin-3. For the last 12 h, cells were incubated with nocodazol to capture cycling cells in G2/M. For each condition, the percentage of cells in each phase (G1-S-G2/M) is indicated. ( d ) U2OS cells were co-transfected with the indicated siRNAs, either with a control anti-miRNA or a specific anti-miR-17/106b pool and analysed as in panel ( b ). ( e ) Cell cycle analysis of U2OS cells transfected as in ( d ) and treated with ionizing radiation. Flow cytometry analysis was performed as in ( c ). All error bars in ( a – e ) represent standard deviation of technical replicates, n =3. Full size image Next, we examined the effect of RBM38 on the p53 response by treating cells with Nutlin-3, a specific inhibitor of the p53–mdm2 interaction. Cell cycle analyses revealed that whereas the response of HCT116 wt to Nutlin-3 was effectively reduced when RBM38 was suppressed (−17% G1), HCT116 ex5−/− cells showed a reduced response (−7% G1) ( Fig. 5c ). As RBM38 counteracts the repression of the miR-17 family on the p21-3′UTR ( Fig. 3e ; Supplementary Fig. S10c ) [35] , we tested whether anti-miR-17 could rescue the loss of p21 induction by DNA damage in RBM38 knockdown U2OS cells. Figure 5d shows that the addition of anti-miR-17/106b pool to cells with RBM38kd largely rescued p21 levels following doxorubicin treatment. Additionally, flow cytometry analysis revealed that whereas loss of RBM38 expression resulted in 12% loss of G1 arrest, inhibition of miR-17/106b activity reduced this effect to 5% ( Fig. 5e ). Thus, our results indicate that RBM38 is required for optimal induction of G1 arrest following DNA damage by shielding the 3′UTRs of prominent p53-target genes from targeting miRNAs. Hypermethylation of RBM38 promoter in p53wt breast tumours Next, we examined RBM38 expression levels in tumours characterized with wt or mutant p53, as RBM38 expression is required for p53 function. In two independent breast cancer cohorts [36] , [37] , we identified a significant reduction in RBM38 mRNA levels in the p53 wild-type subset, when compared with mutant p53 ( Fig. 6a ; P =3.55×10 −9 ; Wilcoxon test). We therefore examined whether CpG methylation could underlie the reduced level of RBM38 in wt p53 breast cancer. Methylation status of CpG islands covering RBM38 promoter region was measured in a cohort of 102 breast cancer tumours, of which 44 harboured mutated p53. Importantly, while RBM38 promoter was methylated in 26% of the p53-wt samples, only 7% of the p53-mutant tumours showed presence of methylation ( Supplementary Table S4 ). Moreover, RBM38 expression was significantly reduced in the subset of samples in which its promoter was found methylated ( Fig. 6b ; P =4.7×10 −3 ; Wilcoxon test), pinpointing the inhibitory influence of methylation on RBM38 expression. To experimentally test the effect of DNA methylation on RBM38 expression, we examined the methylation status of RBM38 CpG islands in several breast cancer cell lines and identified two cell lines (MDA-MB-231 and MDA-MB-436) to be positive ( Fig. 6c,d ). Treatment of these two cell lines with 5-aza-2′-deoxycytidine, a DNA demethylating agent, induced RBM38 expression by at least threefold ( Fig. 6e ). This supports an active silencing mechanism of RBM38 expression by DNA methylation at nearby CpG islands and proposes that this event participates in the tumorigenesis process of wt p53 breast tumours by numbing p53 ability to activate its target genes. 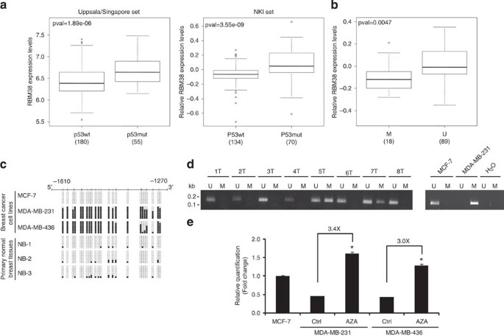Figure 6: CpG island hypermethylation-associated silencing of RBM38 in breast cancer. (a) Comparison between RBM38 expression level in p53-wt and p53-mutant breast cancer samples was carried out in two large and independent cohorts (NKI and Uppsala/Singapore cohorts36,37) for which both expression profile and p53 status data are available. (P-values were calculated using Wilcoxon test). (b) Comparison between RBM38 expression level in breast cancer samples in which its promoter CpG island is methylated (M) and unmethylated (U) (P-values were calculated using Wilcoxon test). (c) Bisulfite genomic sequencing analysis of RBM38 CpG island in human breast cancer cell lines and normal breast (NB) samples. Eight single clones are represented for each case. Locations of CpG dinucleotides (vertical lines) are shown. Presence of unmethylated or methylated CpGs is indicated by white or black squares, respectively. (d) Methylation-specific PCR analyses of RBM38 in primary breast cancer samples. The presence of a band under the U lane indicates unmethylated alleles, while the presence of a band under the M lane indicates methylated alleles. MCF-7 and MDA-MB-231 are shown as negative and positive controls for methylated alleles, respectively. (e) Restored RBM38 expression on treatment with DNA demethylating agent 5-aza-2′-deoxycytidine (AZA) in RBM38 CpG island methylated cell lines. Data represent relative expression (mean±s.d.,n=3 independent experiments, *P<0.05, two-tailed student'st-test) evaluated by RT–qPCR. Figure 6: CpG island hypermethylation-associated silencing of RBM38 in breast cancer. ( a ) Comparison between RBM38 expression level in p53-wt and p53-mutant breast cancer samples was carried out in two large and independent cohorts (NKI and Uppsala/Singapore cohorts [36] , [37] ) for which both expression profile and p53 status data are available. ( P -values were calculated using Wilcoxon test). ( b ) Comparison between RBM38 expression level in breast cancer samples in which its promoter CpG island is methylated (M) and unmethylated (U) ( P -values were calculated using Wilcoxon test). ( c ) Bisulfite genomic sequencing analysis of RBM38 CpG island in human breast cancer cell lines and normal breast (NB) samples. Eight single clones are represented for each case. Locations of CpG dinucleotides (vertical lines) are shown. Presence of unmethylated or methylated CpGs is indicated by white or black squares, respectively. ( d ) Methylation-specific PCR analyses of RBM38 in primary breast cancer samples. The presence of a band under the U lane indicates unmethylated alleles, while the presence of a band under the M lane indicates methylated alleles. MCF-7 and MDA-MB-231 are shown as negative and positive controls for methylated alleles, respectively. ( e ) Restored RBM38 expression on treatment with DNA demethylating agent 5-aza-2′-deoxycytidine (AZA) in RBM38 CpG island methylated cell lines. Data represent relative expression (mean±s.d., n =3 independent experiments, * P <0.05, two-tailed student's t -test) evaluated by RT–qPCR. Full size image Our results portray a model whereby RBM38 potentially inhibits miRNA function on many mRNAs, whereas some mRNAs are selectively spared. This discrimination operates when RBM38 is induced in a p53-dependent manner following DNA damage. Although RBM38 supports the induction of several p53 mRNA targets by relieving miRNA repression, SIRT1, a target of miR-34a, which is a downstream target of p53, is spared ( Fig. 7a ). This allows for differential regulation of gene expression and optimal cell cycle response to DNA damage. Moreover, tumour data analysis revealed a correlation between DNA methylation of the RBM38 promoter region, low RBM38 expression levels, and wt p53 status, suggesting a tumour suppressive role of RBM38 in breast cancer ( Fig. 7b ). 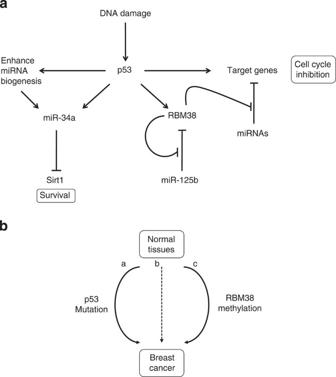Figure 7: A model for RBM38 function and implication in breast cancer. (a) Model for RBM38 function within the p53 pathway. (b) Scheme illustrating possible ways to inactivate or alter (p53 mutation-a, RBM38 methylation-c, other-b) the p53 pathway in breast cancer. Figure 7: A model for RBM38 function and implication in breast cancer. ( a ) Model for RBM38 function within the p53 pathway. ( b ) Scheme illustrating possible ways to inactivate or alter (p53 mutation-a, RBM38 methylation-c, other-b) the p53 pathway in breast cancer. Full size image p53 modulates miRNA production and biogenesis at several levels. It activates global miRNA production by associating with essential components of the miRNA biogenesis machinery. In addition, p53 activates miR-34a to induce growth arrest. Our results unravel an extra layer of miRNA regulation by p53 that relies on the modulation of the activity of specific miRNAs on p53 targets. We show that p53 induces the RNA-binding protein RBM38, which, in turn, limits the accessibility of miRNA sites on the 3′UTRs of its target gene transcripts. In contrast, the SIRT1-3′UTR, a downstream target of miR-34a, is not significantly affected by RBM38. This indicates that selective miRNA-mediated mechanisms act to enhance p53 function. Here we constructed an expression library of RNA-binding proteins, which was subsequently used to identify new RBPs involved in the regulation of miRNA activity. We identified RBM38 as a specific inhibitor of miR-150 function on the c-Myb-3′UTR. Interestingly, the spectrum of action of RBM38 was not limited to miR-150 blocking but included many others ( Fig. 3e ; Supplementary Fig. S6 ). Analogously, our lab previously reported that the RNA-binding protein Dnd1 was able to block the access of miR-206 to Cx43-3′UTR as well as miR-372/373 to LATS2-3′UTR [31] . Despite having a similar function and overlapping targets, Dnd1 and RBM38 seem to have distinct 'raison d'être'. Whereas Dnd1 is specifically expressed in germ cells, RBM38 expression is observed in many human cells and tissues. Furthermore, the RBMS1, 2 and 3 homologues of Dnd1 have similar activity but an entirely different pattern of expression, indicating different roles in cell regulation. A context-dependent change in proteins regulating miRNAs is also observed in miRNA biogenesis, where the processing of let-7 pri-miRNA is tuned by either lin-28 or KSRP protein, two proteins that are expressed in stem and somatic cells, respectively [16] , [18] , [21] , [22] . Altogether, this argues that the specificity of action of miRNA-regulating RBPs is dictated by their expression pattern. Our results indicate that p53 induces the RNA-binding protein RBM38 to influence the expression of several p53-target genes by blocking miRNA accessibility. Shu et al . recently identified RBM38 as a direct target of p53 and linked it to the stability of basal and stress-induced p21 transcripts [29] . Here we confirm this observation and further extend it to other p53-target genes. Some of these genes are targets of miRNAs, and we show that RBM38 effectively counteracted the function of miR-17/106b on the p21-3′UTR, miR-125b on the RBM38-3′UTR, miR-153 on the DDIT4-3′UTR, and miR-372/373 on the LATS2-3′UTR, providing a direct link between RBM38 and activity of specific miRNAs. Interestingly, it has recently been shown that RBM38 and the AU-rich-element-binding protein HuR can physically interact and collaborate to regulate p21 mRNA stability [38] . Bhattacharyya et al . previously demonstrated that during stress HuR translocates from the nucleus to the cytoplasm, where it can bind to the 3′UTR of CAT-1 mRNA and modulate its translation/stability by blocking the miRNA-122 function [23] . However, the importance of the interaction between RBM38 and HuR to their function and target selection remains largely unexplored. Although the statistical targeting of Us in vivo , highlighted by the iCLIP data, predicts that RBM38 targets U-rich sequences, comparison of the functionally equivalent sites on p21 and c-Myb would indicate that the specificity is probably U/G and not U. This partial discrepancy can be explained because of the single-stranded tendency of U-rich sequences, which are, therefore, more available in vivo for proteins targeting single-stranded RNA (ssRNA). Indeed, our in vitro binding assays confirm the in vivo target selectivity of RBM38 RRM domain for p21 and c-Myb. In this context, the iCLIP data confirm the general function and targeting of the protein, but they should not be considered as strictly predictive of the sequences targeted in vivo . Both the absolute affinity and the affinity difference between cognate and non-cognate systems indicate that the RBM38–RNA interactions take place within a multi-component system. We have recently shown that a 20-fold difference in affinity separates a functional and a non-functional interaction in a system regulating the peak in c-Myc transcription during cell cycle. There, the modest affinity difference allows a precise regulation of the length and intensity of the peak of c-Myc concentration. Regulation by RBM38 must also be precise, and the modest affinity difference between cognate and non-cognate RNAs is probably necessary to guarantee a precise and reversible switch of p21 post-transcriptional regulation. Such regulatory mechanisms are typically found in multi-component systems. This is consistent with the intermediate affinity of RBM38 for the specific miRNA target region, which is typical of the interaction between an isolated RNA-binding domain and ssRNA in multi-component complexes. In vivo , the RBM38 RRM–RNA binding affinity is likely to be boosted by simultaneous interaction of other RNA-binding proteins with the RNA target, RBM38 oligomerization or the general structural context [38] . Functional impairment of the p53 pathway is instrumental for tumour progression. Whereas the p53 pathway is inactivated in most, if not all, cancers, the p53 gene is generally mutated in about 50% of tumours. However, certain tumours, such as breast and prostate, show much lower frequency of mutations in p53. In those tumours, other alterations in the p53 pathway occur that weaken p53 tumour-suppressive activity. Here we propose that RBM38 is important for full p53 function, and that its level of expression correlated with wt p53 status. The fact that a significant proportion of wt p53 tumours possess DNA methylation of RBM38 promoter region suggests an active mechanism to silence RBM38 in those tumours. Constructs Coding sequences were PCR amplified using cDNA pools derived from various cell lines and subsequently cloned to pcDNA5/FRT/V5-His TOPO (Invitrogene). All UTR sequences were obtained from human genomic DNA PCRs and cloned downstream of the Renilla luciferase ( Xho 1/ Not 1) in psiCHECK2 vector. RBM38 knockdown constructs were cloned in pRETROSUPER. p53 knockdown construct has been previously described [39] . For the iCLIP, RBM38 ORF was cloned ( Bam H1- Asc 1) in pcDNA3pQE vector, downstream of two streptavidin and one Histidine tags. To generate a RBM38-HA-inducible cell line, we carboxy-terminally fused the HA epitope (YPYDVPDYA) to RBM38 ORF and cloned ( Sal 1) the coding sequence in the previously described tetracycline-dependent lentiviral vector [40] . All primers used to PCR amplify wild-type/mutant RBPs and UTRs as well as shRNA and siRNA sequences are listed in Supplementary Table S1 . Cell culture and transfection HCT116 cells were grown in RPMI and HeLa, U2OS, MCF-7, ZR-75.1, MDA-MB-231 and MDA-MB-436 were cultured in DMEM containing 10% FBS, penicillin and streptomycin at 37 °C and 5% CO 2 . The screening was setup in a 384-well plate format and performed by reverse-transfecting U2OS cells with 5 ng of psiCHECK2-c-Myb, 10 ng of miRNA and 60 ng of each RBP using fugene (Roche). Hits validation, luciferase assays and overexpression/knockdown (pRETROSUPER) experiments were conducted using fugene. RNAi experiments were carried out using Dharmafect transfection reagent-1 and between 5 to 100 nM of siRNA: Scramble (AUUCGUGAGGCAGAAGCGA), RBM38-1 (UGAGAGGGCUUGCAAAGAC), RBM38-2 (GACACCACGUUCACCAAGA) and RBM38-3 (ACGCCUCGCUCAGGAAGUA), RBM38-4 (CGUGAACCUGGCAUAUCUG), RBM38-5 (CACCUUGAUCCAGCGGACUUA), with or without anti-hsa-miR-17 (AM10198, Ambion) and anti-hsa-miR106b (AM10067, Ambion) or hsa-miR-17 duplex (CAAAGUGCUUACAGUGCAGGUAG). To induce a p53 stress-response, cells were treated with 0.4 μg ml −1 of doxorubicin (D1515, Sigma), 4–8 μM of Nutlin-3 (N6287, Sigma) or 15 Gy of ionizing radiation for 24 h. Inducible GFP and RBM38-HA cell lines were generated using a tetracycline-dependent lentiviral vector, as previously described [40] . For epigenetic drug treatments, cells were treated with 2 μM 5-aza-2′-deoxycytidine (A3656, Sigma) for 72 h. Protein analysis Whole-cell lysates were prepared using Urea lysis buffer (6 M Urea, 2% SDS and 50 mM Tris–HCl pH 6.8) and sonication. Protein extract concentrations were assessed using the DC protein assay (Bio-Rad). Before electrophoresis, protein samples were mixed with laemmli buffer 4×, boiled, SDS/PAGE-resolved and transferred on PVDF membranes. Protein detection was performed using primary antibodies recognizing p53 (DO1, Santa Cruz, 1:1,000), p21 (Sc-397, Santa Cruz, 1:1,000), CDK4 (Sc-260, Santa Cruz, 1:1,000), RBM38 (18-003-43641, GenWay, 1:2,000), Ago2 (C34C6-Cell Signaling and ab32381-Abcam, 1:1,000 and 1:300 for IP), V5 (R960-25, Invitrogen, 1:5,000), HA (sc-805/Y-11, Santa Cruz, 1:1,000, 1:500 for IF and 1:200 for IP), GFP (A6455, Invitrogen, 1:1,000) and tubulin (Sc-8035, Santa Cruz, 1:1,000). Membranes were further incubated with the appropriate secondary antibodies (Dako) and proteins were visualized using ECL reagents (GE Healthcare). For in vitro binding assays, RBM38wt or mutant protein (amino acids 23–110, NP_055096) was expressed as a TEV protease-cleavable amino-terminal HisTag in E.coli strain BL21 (DE3) using a pETM-11 vector (EMBL-Heidelberg, Protein Expression Facility). 15 N and 15 N 13 C-labelled protein was expressed and purified as reported [41] . Briefly, the tagged protein was purified from the soluble fraction of the cell lysate by nickel-affinity chromatography (Qiagen) and the His-tag removed by overnight TEV protease digestion at 4 °C, followed by a second nickel affinity step. The RBM38 was further purified by gel filtration (Superdex 75 16/60 column, Pharmacia) and finally dialysed overnight against the final buffer, 10 mM Tris–HCl pH 7.4, 100 mM NaCl. Protein purity as assessed by SDS–PAGE and Coomassie staining was >95%. The protein was concentrated to 0.6–0.7 mM and stored in 10 mM Tris–HCl pH 7.4, 100 mM NaCl, 2 mM TCEP, 0.05% (w/v) NaN 3 at −20 °C. RNA analysis Total RNA was isolated using TRIzol reagent (Invitrogen). After reverse transcription using oligo dT and SuperScriptII (SSII) reverse transcriptase (Invitrogen), real-time quantitative PCR analysis was performed using gene-specific primers: RBM38 Fwd (5′-AAGACCCGAACCCCATCATC-3′) Rev (5′-CACGATGGCTGGTGGGTAGA-3′), p21 Fwd (5′-TACCCTTGTGCCTCGCTCAG-3′) Rev (5′-GAGAAGATCAGCCGGCGTTT-3′), GAPDH Fwd (5′-TGCACCACCAACTGCTTAGC-3′) Rev (5′-GGCATGGACTGTGGTCATGAG-3′) and SYBR Green PCR master mix (Applied Bioystems). Mature hsa-miR-17, hsa-miR-22, hsa-miR-34a, hsa-miR-107, hsa-miR-150, hsa-miR-200c, hsa-miR-222 and hsa-miR-429 were quantified using Taqman microRNA detection assay (Applied Biosystems). The 18S ribosomal RNA or GAPDH were used as an internal control for real-time PCRs. RNase protection assays for miR-150 were performed using the Hybspeed RPA and mirVana kits (Ambion) according to the manufacturer's instructions and the primer 5′-GGCGGCTCCTCTCCCCATGGCCCTGTCTCCCAACCCTTGTACCAGTGttttcctgtctc-3′. Cyclophilin probe contained nucleotides 46–149 of Accession # BC013915. All reactions were carried out using 2 μg of RNA extracted from the nuclear and cytoplasmic fractions obtained using the NE-PER Nuclear and Cytoplasmic Extraction Reagents (Pierce). Flow cytometry Cells were arrested in mitosis using 250 ng ml −1 nocodazole for 12 h. Cells were then trypsinized, washed and resuspended in PBS containing 0.6% NP-40, 50 mg ml −1 RNaseA and 50 mg ml −1 propidium iodide for 10 min. Cell cycle profiles were visualized using FACScan and the Cell Quest software (Becton Dickinson). NMR spectroscopy All NMR samples ( 15 N- and 15 N 13 C-labelled RBM38) were prepared in 90% H 2 O/10% H 2 O solutions of 10 mM Tris–HCl pH 7.4, 100 mM NaCl, 2 mM TCEP at 0.05–0.7 mM protein concentration. The NMR spectra were recorded at 37 or 27 °C on Varian Inova and Bruker Avance spectrometers equipped with cryoprobes and operating at 600, 700 and 800 MHz 1 H frequencies. The spectra were processed with the NMRPipe package [42] and analysed using Sparky. Backbone assignment of RBM38 at 37 °C was obtained from the analysis of HNCACB, CBCA(CO)NH and HNCO experiments as described in refs 43 and 44 . In vitro binding analysis Chemically synthesized (Thermo Scientific) RNA 22-mers recapitulating c-Myb, p21 and SIRT1 miRNA-binding sites were titrated into 25 or 50 μM sample of 15 N- labelled RBM38 in 10 mM Tris–HCl pH 7.4, 100 mM NaCl, 2 mM TCEP and the recommended amount of RNasin (Promega). Protein–RNA binding was monitored by recording 15 N 1 H correlation spectra at 0:1, 0.5:1, 1:1, 2:1, 4:1 and 8:1 RNA:protein ratios and measuring chemical shift changes of six resonances in fast exchange regime on an NMR timescale. The averaged chemical shift change of the resonances was calculated using the equation Δδ avg =((Δδ N /10) 2 +Δδ H 2 ) 1/2 and was plotted against the RNA:protein ratio to obtain the binding isotherms. Binding constants were obtained using the program xcrvfit (Sykes Laboratory) assuming a single site of binding. iCLIP The procedure used for the iCLIP has been previously described [33] . A total of 13,386 binding sites were mapped to validated protein-coding transcripts. Search for binding site signature was done using the AMADEUS de-novo motif discovery package [45] . Over-represented motifs were searched in the binding-site regions (defined as the 16-nt-long regions centred at the location mapped by iCLIP as the binding nucleotide) compared with their flanking sequences of the same length and on both sides of the binding region. RNA immunoprecipitation GFP and RBM38-HA clones were induced with Doxycycline (1 μg ml −1 for 24 h) and treated with Nutlin-3 (8 μM for 12 h). Before lysis, cells were crosslinked 15 min with 1% formaldehyde, inactivated with 330 mM glycine, washed with PBS and resuspended in lysis buffer (50 mM Hepes pH 7.5, 150 mM NaCl, 1% Triton X-100, 0.1% Sodium deoxycholate) supplemented with protease inhibitor mixture (Roche), RNaseOUT (Invitrogen) and 1 mM dithiothreitol. The extracts were then sonicated, insoluble materials discarded and protein concentrations assessed. For each condition, Ago2 was immunoprecipitated from 2 mg of cell extract using 2 μg of antibody and Gammabind G sepharose (GE Healthcare) beads preblocked with 5% BSA. Extracts were incubated 5 h in a tumbler placed at 4 °C. After extensive washing, reverse crosslinking was performed 5 h at 70 °C and RNA was extracted (Trizol, Invitrogen) to be subjected to RT–qPCR. Fluorescence microscopy Microscope cover slips were placed in polylysine-coated six-well culture dishes. The cells were then plated at a density of 5×10 5 cells per well and allowed to adhere for 24 h before induction (Doxycycline, 1 μg ml −1 ). Cells were fixed with 3% formaldehyde and subsequently permeabilized with PBS-Triton X-100 (0.3%) solution. After blocking 1 h with 2% PBS-Milk, the HA epitope was detected using the aforementioned primary antibodies and the Alexa Fluor 488 Dye-conjugated secondary antibody. Images were captured using an AxioCam MRc CCD camera (Carl Zeiss Microimaging). Microarray analysis Expression profiles were recorded in independent duplicates using Illumina WG6v3 arrays containing more than 49 K probes. Expression levels were calculated using Illumina's BeadStudio package. Only probes flagged as 'Present' (detection P -value <0.05) in at least two out of the eight arrays were used for subsequent analysis (24,630 probes). Arrays were normalized using quantile normalization. Expression dataset was then analysed using the EXPANDER package [46] . Probes that responded to doxorubicin treatment by at least a factor of 2.0 were subjected to k-means cluster analysis (2,990 probes). GO enrichment analysis was carried out using TANGO. The microarray data has been deposited in the Gene Expression Omnibus (GEO) database under accession code GSE32301. DNA methylation analysis CpG islands were identified in silico using Methyl Primer Express v1.0 software. DNA methylation status was established by bisulfite genomic sequencing of multiple clones or methylation-specific PCRs in DNA samples previously treated with sodium bisulfite (EZ DNA methylation Gold kit, Zymo Research). The primers used are listed in Supplementary Table S1 . Accession codes: The microarray data has been deposited in the Gene Expression Omnibus (GEO) database under accession code GSE32301 . How to cite this article: Léveillé, N. et al . Selective inhibition of microRNA accessibility by RBM38 is required for p53 activity. Nat. Commun. 2:513 doi: 10.1038/ncomms1519 (2011).